Chiral spin torque arising from proximity-induced magnetization Domain walls can be driven by current at very high speeds in nanowires formed from ultra-thin, perpendicularly magnetized cobalt layers and cobalt/nickel multilayers deposited on platinum underlayers due to a chiral spin torque. An important feature of this torque is a magnetic chiral exchange field that each domain wall senses and that can be measured by the applied magnetic field amplitude along the nanowire where the domain walls stop moving irrespective of the magnitude of the current. Here we show that this torque is manifested when the magnetic layer is interfaced with metals that display a large proximity-induced magnetization, including iridium, palladium and platinum but not gold. A correlation between the strength of the chiral spin torque and the proximity-induced magnetic moment is demonstrated by interface engineering using atomically thin dusting layers. High domain velocities are found where there are large proximity-induced magnetizations in the interfaced metal layers. The manipulation of domain walls by spin-polarized currents allows for novel memory [1] , [2] and logic [3] devices that were not previously possible by using magnetic fields alone. Early studies on the current-driven motion of domain walls (DWs) in both in-plane [4] , [5] , [6] , [7] , [8] and thick, perpendicularly magnetized Co/Ni nanowires [9] could be well understood by the phenomenon of volume spin-transfer torque (V-STT) [10] , [11] , [12] that arises from the transfer of spin angular momentum from spin-polarized current in the interior of the magnetic material to the local magnetization [10] , [11] . Much higher DW velocities were subsequently reported in ultrathin ferromagnetic layers displaying large perpendicular magnetic anisotropy (PMA) [13] , [14] , [15] that are difficult to reconcile with V-STT. Furthermore, the DWs move in the direction of current, opposite to that expected from conventional V-STT [13] , [14] , [15] , [16] . Two mechanisms that were initially proposed to account for this unexpected behaviour, based on Rashba magnetic fields at magnetic/oxide interfaces [17] , [18] , [19] , and on spin accumulation derived from spin currents generated through the spin Hall effect (SHE) [20] , [21] in platinum underlayers (ULs) [22] , cannot alone account for the observed current induced motion of the DWs in PMA nanowires [15] . Recently, it has been shown experimentally that in perpendicularly magnetized Co/Ni/Co stacks grown on Pt layers, in which the DWs move very fast, the DWs are subject to large internal effective fields directed along the nanowire, which alternate in direction between successive DWs [15] . These internal fields cause the most stable DW structure to be a Néel structure, in which the magnetization rotates in a plane parallel to the length of the nanowire, rather than a Bloch structure, and, moreover, establish that all the DWs in the wire have the same chirality. The combined effect of these internal fields together with SHE-generated spin currents gives rise to a chiral spin torque (CST) that is responsible for the high velocity of DWs along the current direction in Pt/Co/Ni/Co nanowires [15] , [23] , [24] , [25] . The origin of the internal fields responsible for the CST has been speculated to be derived from a Dyzaloshinskii–Moriya interaction (DMI) [15] , [26] , [27] , [28] , [29] , [30] , [31] at the Pt/Co interface. However, the DMI originates from spin–orbit coupling (SOC) that is large in Pt but much weaker in Co and Ni, and the mechanism by which the DMI can generate such large internal fields at the DWs in the Co/Ni/Co magnetic trilayer is not understood. Here we show that the CST is not limited to Pt ULs but is found for other heavy metal ULs including Pd and Ir, but not Au. We find that the strength of the internal effective fields in these different systems is consistent with their originating from a DMI. Moreover, we show that the CST is only observed when the magnetic trilayer is in contact with metals that display a proximity-induced magnetic moment (PIM), thus shedding new light on the mechanism underlying the CST in these systems. Underlayer dependence of current induced domain wall motion Nanowires were formed from magnetic sandwiches of (3 Å Co/7 Å Ni/ 1.5 Å Co) deposited on metallic ULs of Pd, Ir, Pt and Au. Only structures that exhibited perpendicular magnetic anisotropy (PMA) with square magnetic hysteresis loops were used for these studies. The current-induced motion of individual DWs was studied in nanowires 2 μm wide and 50 μm long ( Fig. 1a ) that were fabricated by optical lithography and argon ion mill etching. Kerr optical microscopy (see Methods for details) was used to track the motion of individual domain walls along the nanowires in response to nanosecond long current pulses. Typical examples of Kerr images that were used to determine the direction and velocity of the DW motion in Co/Ni/Co nanowires on Ir and Au ULs, respectively, are shown in Fig. 1b,c . The dependence of DW velocity on the current density J is shown in Fig. 1d–g for [Co/Ni/Co] nanowires grown on Pd, Ir, Pt and Au, respectively, for current pulses varying in length from 5 to 100 ns. In each case, the DWs only move above a threshold current density J C that increases the shorter is the current pulse length. J C varies significantly with the UL metal, as does the maximum DW velocity, which is much smaller for Pd and Ir than for Pt. For Pd, Ir and Pt ULs the DWs move in the direction of the current flow, whereas, by contrast, for ULs formed from Au the DWs move in the opposite direction along the electron flow. For all four metal ULs, however, all the DWs, whether up/down (↑↓) or down/up (↓↑), move at the same speed and in the same direction. 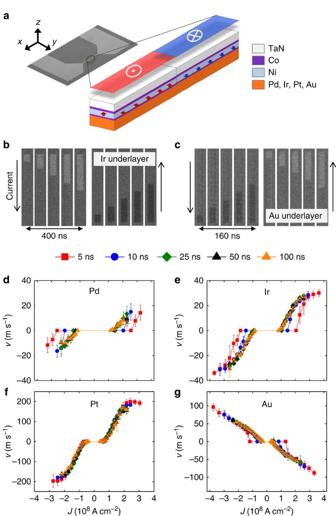Figure 1: Dependence of current-driven DW motion in Co/Ni wires on underlayer. (a) Schematic representation of a device showing a UL/ 3 Co/7 Ni/1.5 Co stack grown on various ULs and two magnetic domains in which the magnetization is perpendicular to the plane of the wafer: red and blue correspond to magnetization pointing out of or into the plane, respectively. (b,c) Kerr microscopy images of a single DW moving along a nanowire in response to sequences of current pulses (J~\n3.0 × 108A cm−2) composed of ten 10-ns and eight 5-ns long pulses. Typical images are shown for Ir and Au ULs, respectively, for positive and negative current polarities, as indicated by the arrows. Note that the lighter and darker contrast corresponds to up and down magnetization directions, respectively. (d–g) DW velocities as a function of the current pulse densityJfor 50 Pd, 30 Ir, 50 Pt and 30 Au ULs. The current pulse lengths are varied from 5 ns (red squares), 10 ns (blue circles), 25 ns (green diamonds), 50 ns (black triangles), to 100 ns (orange triangles), respectively. The error bars in all figures correspond to one s.d. All thicknesses are given in Å. Figure 1: Dependence of current-driven DW motion in Co/Ni wires on underlayer. ( a ) Schematic representation of a device showing a UL/ 3 Co/7 Ni/1.5 Co stack grown on various ULs and two magnetic domains in which the magnetization is perpendicular to the plane of the wafer: red and blue correspond to magnetization pointing out of or into the plane, respectively. ( b , c ) Kerr microscopy images of a single DW moving along a nanowire in response to sequences of current pulses ( J ~\n3.0 × 10 8 A cm −2 ) composed of ten 10-ns and eight 5-ns long pulses. Typical images are shown for Ir and Au ULs, respectively, for positive and negative current polarities, as indicated by the arrows. Note that the lighter and darker contrast corresponds to up and down magnetization directions, respectively. ( d – g ) DW velocities as a function of the current pulse density J for 50 Pd, 30 Ir, 50 Pt and 30 Au ULs. The current pulse lengths are varied from 5 ns (red squares), 10 ns (blue circles), 25 ns (green diamonds), 50 ns (black triangles), to 100 ns (orange triangles), respectively. The error bars in all figures correspond to one s.d. All thicknesses are given in Å. Full size image Influence of longitudinal field on domain wall velocity To explore the origin of the CST, we compare the dependence of the DW velocity v (measured at J =2 × 10 8 A cm −2 ) on a longitudinal magnetic field H x applied along the nanowire for Co/Ni/Co sandwiches prepared on Pd, Ir, Pt and Au ULs in Fig. 2a,c,e,g . Data are shown for both ↑↓ and ↓↑ DWs (red and blue symbols, respectively) and for positive and negative currents (open and closed symbols, respectively). For Pd, Ir and Pt ULs the dependence of v on H x has two important characteristics. First, v increases almost linearly with H x except for an offset close to H x ~\n0 that is more clearly visible for the samples with Pd and Ir ULs. Second, the DW velocity becomes zero at a critical value of H x that we will name the crossing field, H CR . H CR has the same magnitude but the opposite sign for ↑↓ and ↓↑ DWs. The behaviour for Pd, Ir and Pt is similar to that which we reported previously for various Co/Ni/Co stacks grown on Pt [15] . In contrast, the data shown in Fig. 2g for a Au UL are clearly very different and there is almost no dependence of v on H x . Note that the maximum value of H x that can be accessed is limited by the threshold field above which DWs are nucleated that is proportional to , where K is the perpendicular magnetic anisotropy constant and M S is the saturation magnetization: thus, for Au, and to a lesser extent Pd ULs, significantly smaller values of H x can be applied than for Pt and Ir ULs. 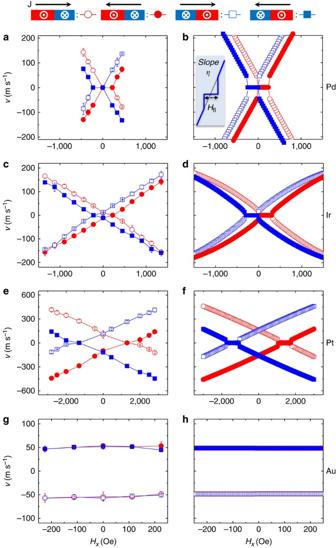Figure 2: Dependence of current-driven DW dynamics on underlayer. (a,c,e,g) Measured DW velocity versusHx, and (b,d,f,h) corresponding 1D model calculations for UL/ 3 Co/7 Ni/1.5 Co wires with 50 Pd, 30 Ir, 15 Pt and 30 Au ULs, respectively forJ~\n2 × 108A cm−2. Red and blue symbols represent ↑↓ and ↑↓ DWs, respectively. Open and solid symbols correspond to positive (+x) and negative (−x) current directions, respectively. Key fitting parameters used in the 1D model are summarized along with key experimentally determined parameters inTable 1. (See details inSupplementary Table 1). The error bars in (a,c,e,g) correspond to one s.d. All thicknesses are in Å. The inset inbshows the definitions ofηandHfl. Figure 2: Dependence of current-driven DW dynamics on underlayer. ( a , c , e , g ) Measured DW velocity versus H x , and ( b , d , f , h ) corresponding 1D model calculations for UL/ 3 Co/7 Ni/1.5 Co wires with 50 Pd, 30 Ir, 15 Pt and 30 Au ULs, respectively for J ~\n2 × 10 8 A cm −2 . Red and blue symbols represent ↑↓ and ↑↓ DWs, respectively. Open and solid symbols correspond to positive (+ x ) and negative (− x ) current directions, respectively. Key fitting parameters used in the 1D model are summarized along with key experimentally determined parameters in Table 1 . (See details in Supplementary Table 1 ). The error bars in ( a , c , e , g ) correspond to one s.d. All thicknesses are in Å. The inset in b shows the definitions of η and H fl . Full size image The dependence of v on H x shown in Fig. 2a,c,e,g can be well understood within the 1D model (see Supplementary Note 1 and Supplementary Fig. 1 ), using the fitting parameters given in Table 1 . As shown in the schematic diagram in the inset to Fig. 2b , there is a range of H x over which v varies approximately linearly with H x with a slope that is given by , where γ is the gyromagnetic ratio, Δ is the DW width, H SHE is the effective field derived from the SHE, α is the Gilbert damping parameter and H k is the DW in-plane shape anisotropy field ( (ref. 32 ), where t is the ferromagnetic layer thickness). Note that H k favours a Bloch DW for the wires used here. The sign of η depends on the DW configuration (− for ↑↓ and+for ↓↑). The magnitude of η varies in the order, Pd>Ir>Pt, largely due to the variation in Δ ( ) that varies in the inverse order, Pd>Ir>Pt (see Table 1 ). Note that η depends only weakly on H SHE . Near H x = H CR there is a discontinuity in the variation of v with H x that may be accounted for by including in our 1D model static pinning of the DW (see Supplementary Note 1 and Supplementary Fig. 2 ). We define a window in H x , centred around H CR of width H fl for which we find the DW velocity is zero, given by (see inset to Fig. 2b ). Table 1 Summary of film magnetic properties and 1D model fitting parameters. Full size table The spin Hall angle θ SHE can be derived from H SHE , as discussed in the Supplementary Note 1 . As shown in Table 1 , Pt displays the largest value of θ SHE which is about two times that exhibited by Pd. θ SHE in Ir is much smaller. These values are in reasonable agreement with experimental results [22] , [33] , [34] and theoretical predictions [35] . The data for Au ULs clearly show that there is no SHE for Au ULs and consequently no CST in this case. Influence of Au dusting layers on domain wall dynamics The strong dependence of the DW velocity on H x not only reflects the important role of the SHE but, most importantly, the crossing field where the DW velocity goes to zero is a direct manifestation of an internal effective magnetic field, as discussed above. The fact that Pd, Ir and Pt all exhibit a crossing field suggests a common mechanism of current-induced DW motion for these metals. To further explore the origin of the crossing field we introduce ultrathin ‘dusting’ layers of Au at the UL/Co interface in the magnetic stacks. For Au layers even just 1 or 2 Å thick, as shown in Fig. 3a,b , the crossing field is markedly reduced and the role of the static DW pinning becomes more pronounced for all three ULs. The detailed dependence of H CR , H fl and η are shown in Fig. 3c–e and discussed in more detail in the Supplementary Information. The DW velocity is decreased to zero for Au layers with thicknesses below ~\n4 Å in each case ( Fig. 3f ). Associated with changes in the DW velocity are significant changes in magnetization and magnetic anisotropy of the film stacks, as detailed in Fig. 3g,h . All the stacks remain perpendicularly magnetized for all Au layer thicknesses, although K eff drops substantially for Pt and Ir ULs, but the changes are much smaller for Pd ULs. Perhaps, most interestingly, for all three ULs the magnetization is much reduced, by a quantity δM S , with the introduction of the Au dusting layers, which we associate with the elimination of a PIM in the ULs that is induced by an exchange interaction with the neighbouring Co layer: δM S is very large and ranges from 19 to 29% of M S (see Table 1 ). 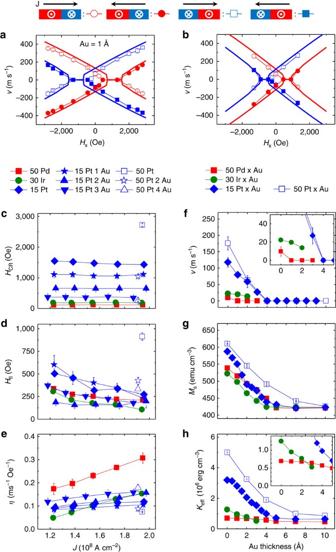Figure 3: Role of proximity-induced magnetization in underlayer. An ultra-thin Au spacer layer is inserted between the UL (50 Pd, 30 Ir, 50 Pt, and 15 Pt) and the Co/Ni/Co stack. (a,b) Measured DW velocities versusHxfor 15 Pt/1 Au and 15 Pt/ 2 Au ULs, respectively (J~\n2 × 108A cm−2). Red and blue symbols represent ↑↓ and ↓↑ DWs, respectively. Open and solid symbols correspond to positive and negative currents. The 1D model fitted curves are plotted as solid lines. The error bars correspond to one s.d. (c–e),HCR,HflandηversusJ; 50 Pd (red square), 30 Ir (green circle), 15 Pt (blue diamond), 15 Pt/1 Au (blue star), 15 Pt/2 Au (blue up triangle), 15 Pt/3 Au (blue down triangle), 50 Pt (blue open square), 50 Pt/2 Au (blue open star) and 50 Pt/4 Au (blue open triangle). The error bars inc,dare s.e. values from the least square fits, while those inecorrespond to one s.d. (f–h) Dependence ofν,MSandKeffon Au layer thickness (J~\n2 × 108A cm−2):MSandKeffare obtained from magnetization measurements on unpatterned films: 50 Pd/xAu (red squares), 30 Ir/xAu (green circles), 15 Pt/xAu (solid blue diamonds) and 50 Pt /xAu (open blue squares). The error bars correspond to one s.d. All thicknesses are in Å. For clarity the insets infandhshow an expanded view of the lowxdata. Figure 3: Role of proximity-induced magnetization in underlayer. An ultra-thin Au spacer layer is inserted between the UL (50 Pd, 30 Ir, 50 Pt, and 15 Pt) and the Co/Ni/Co stack. ( a , b ) Measured DW velocities versus H x for 15 Pt/1 Au and 15 Pt/ 2 Au ULs, respectively ( J ~\n2 × 10 8 A cm −2 ). Red and blue symbols represent ↑↓ and ↓↑ DWs, respectively. Open and solid symbols correspond to positive and negative currents. The 1D model fitted curves are plotted as solid lines. The error bars correspond to one s.d. ( c – e ), H CR , H fl and η versus J ; 50 Pd (red square), 30 Ir (green circle), 15 Pt (blue diamond), 15 Pt/1 Au (blue star), 15 Pt/2 Au (blue up triangle), 15 Pt/3 Au (blue down triangle), 50 Pt (blue open square), 50 Pt/2 Au (blue open star) and 50 Pt/4 Au (blue open triangle). The error bars in c , d are s.e. values from the least square fits, while those in e correspond to one s.d. ( f – h ) Dependence of ν , M S and K eff on Au layer thickness ( J ~\n2 × 10 8 A cm −2 ): M S and K eff are obtained from magnetization measurements on unpatterned films: 50 Pd/ x Au (red squares), 30 Ir/ x Au (green circles), 15 Pt/ x Au (solid blue diamonds) and 50 Pt / x Au (open blue squares). The error bars correspond to one s.d. All thicknesses are in Å. For clarity the insets in f and h show an expanded view of the low x data. Full size image The crossing field depends weakly on current density for ULs formed from Pd, Ir and Pt as well as these same ULs with Au dusting layers (when ). This is the most important characteristic feature of the crossing field. Within the 1D model, since there is a contribution to H CR from the V-STT [7] , [36] that increases linearly with J , we conclude that the V-STT contribution to H CR is small. For the Co/Ni/Co stacks used here, this contribution, for J ~\n2 × 10 8 A cm −2 , is ~\n140, ~\n240 and ~\n400 Oe for Pd, Ir and Pt based stacks, respectively (see Supplementary Fig. 3 ), in each case decreasing the intrinsic crossing field, (that is, H CR in the absence of V-STT). Also, as anticipated within the 1D model (see Supplementary Fig. 2 ), as J is increased, pinning can be more easily overcome leading to reduced H fl . Finally, η is only weakly dependent on J for Pt and Pt/Au ULs, for which cases H SHE is large compared with H k , but increases with J for Ir and Pd ULs where, by contrast, H SHE is small compared with H k for small J . Thus, the dependence of η on J is consistent within the 1D model with a J independent θ SHE , as expected. Moreover, θ SHE is not much affected by the introduction of the Au dusting layers, thereby showing that the spin currents generated in the Pd, Ir and Pt ULs, via a SHE, can pass across the Au layers with little attenuation [37] (see Supplementary Table 1 for the case of Pt/Au/Co). We finally discuss the origin of H CR and its relationship with the magnetic properties of the different stacks. Assuming that the J -independent offset field is associated with a DMI, we postulate that H CR will be proportional to the quantity . Our rationale is as follows: first, the DMI originates from the UL/Co interface that also determines the PMA in these stacks. Both the DMI and the PMA are, in a first approximation, proportional to the strength of spin-orbit coupling (SOC), and thus the DMI should be proportional to K [29] , [38] , [39] . Second, since the DMI exchange energy density within the DW can be written as, , where D is a vector that reflects the strength and chirality of the DMI [30] , it follows that , which, since means that . Third, we postulate that the DMI is also proportional to the PIM since the introduction of Au dusting layers eliminates the PIM but not the SHE. 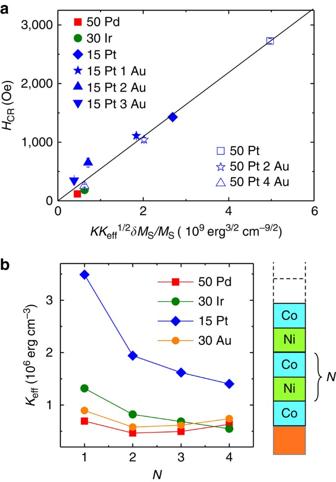Figure 4: Correlation between DMI and perpendicular anisotropy/ induced moment. (a) The crossing fieldHCRis plotted versusfor various ULs. The black solid line is a linear fit to the data that is constrained to pass through zero. Here, the error bars correspond to those forHCR. (b)Keffas a function of N for [Co/Ni]Non various ULs, where N is varied from 1 to 4. Error bars correspond to one s.d. All thicknesses are given in Å. Figure 4a shows that H CR increases in approximate proportion to the quantity consistent with our conjecture. Thus, we propose that the origin of the DMI is closely related to the PIM. In this regard, it is very interesting that the Au/Co and Pd/Co interfaces display very similar values of K and K eff so that, as shown in Fig. 3h , there is very little change in K eff for Pd ULs when Au dusting layers are introduced. This is further supported by the similar dependence of K eff on the number of Co/Ni bilayers in UL/Co/[Ni/Co] N /TaN stacks as shown in Fig. 4b for Au and Pd ULs, whereas there is a much stronger dependence of K eff for Ir and Pt ULs. Thus, one would anticipate a similar magnitude of the DMI for Au and Pd ULs that we do not find. The only distinction between Au and Pd ULs is the PIM, which we therefore argue is a critical ingredient in establishing significant values of DMI. Figure 4: Correlation between DMI and perpendicular anisotropy/ induced moment. ( a ) The crossing field H CR is plotted versus for various ULs. The black solid line is a linear fit to the data that is constrained to pass through zero. Here, the error bars correspond to those for H CR . ( b ) K eff as a function of N for [Co/Ni] N on various ULs, where N is varied from 1 to 4. Error bars correspond to one s.d. All thicknesses are given in Å. Full size image Sample preparation The films used in these experiments were deposited by magnetron sputter deposition at ambient temperature on Si(100) substrates covered with amorphous SiO 2 . A colourized optical micrograph of a typical device is shown in Fig. 1a . The wire in the central portion, where DW motion was imaged, is connected at both ends to wider regions that are used as bond pads for electrical connections. In most cases, we find that the PMA is significantly reduced at the wire bonds, such that DWs are nucleated near the bonds and can propagate in the wire under an external field (cartoon in Fig. 1a ). Once a single DW is injected in the wire, the field is reduced to zero and DW motion is studied by applying a series of current pulses of length t P to the device. Measurement of DW velocity Kerr optical microscopy in differential mode is used to monitor the position of the DW along the nanowire in response to a series of current pulses ( Fig. 1b ). The sensitivity of this technique is sufficient to detect the motion of single DWs in nanowires as narrow as ~\n100 nm. Images are taken after a fixed number of current pulses chosen such that the DW has moved by a significant distance, typically ~\n1–2 μm. The DW velocity is then determined by assuming that the DW moves only during the current pulses. We use a linear fit of the DW position versus the integrated current pulse length t CP, that is, the product of t P and the number of pulses applied. In some cases, the DW may be pinned by a local defect until enough pulses are applied to dislodge it. In these cases, we fit only the portions of the curve in which the DW position depends linearly on t CP . The s.d. of the differential velocity, that is, the point by point derivative of the DW position versus t CP curve, is used to determine an error bar. Note that we define the DW velocity to be positive (negative) when the DWs move along the current (against) flow. DWs move over the entire length of the device at constant velocity, thus excluding driving mechanisms based on irreversible transformations of the DWs. J is calculated from the device resistance by assuming uniform conduction in the metallic layers. DW motion takes place when J exceeds a critical value J C . As shown in Fig. 1d–g , J C decreases significantly for longer current pulses as thermally activated processes become more important [5] . Above J C , the DW velocity increases rapidly with J . Motion at higher current densities is hindered by the random nucleation of reversed domains due to the combined action of STT, Joule heating and the Oersted field from the current. Determination of magnetic anisotropy values The magnetic anisotropy constants K and K eff are determined by measuring the easy-axis and hard-axis magnetic hysteresis loops. When the easy axis component of magnetization ( M z ) is measured as a function of the magnetic field H z applied along the easy axis ( z ), the hysteresis loop is rectangularly shaped (see Supplementary Fig. 4 ). At high enough H z , M z equals the bulk saturation magnetization M S . In contrast, the hard axis component of magnetization ( M x ) increases linearly with H x when the field is applied along the hard axis x ( Supplementary Fig. 4 ). When H x equals the anisotropy field, H eff , M x = M S , then, it follows that, H eff =2 K / M S −4π M S . Hence K = K eff +2π M S 2 and K eff = H eff M S /2. Supplementary Fig. 5 shows typical easy and hard axis magnetization loops for samples with Ir, Pd, Pt and Au underlayers from which K and K eff have been deduced. How to cite this article: Ryu, K.-S. et al . Chiral spin torque arising from proximity-induced magnetization. Nat. Commun. 5:3910 doi: 10.1038/ncomms4910 (2014).